Crystal structures of interleukin 17A and its complex with IL-17 receptor A The constituent polypeptides of the interleukin-17 family form six different homodimeric cytokines (IL-17A–F) and the heterodimeric IL-17A/F. Their interactions with IL-17 receptors A–E (IL-17RA–E) mediate host defenses while also contributing to inflammatory and autoimmune responses. IL-17A and IL-17F both preferentially engage a receptor complex containing one molecule of IL-17RA and one molecule of IL-17RC. More generally, IL-17RA appears to be a shared receptor that pairs with other members of its family to allow signaling of different IL-17 cytokines. Here we report crystal structures of homodimeric IL-17A and its complex with IL-17RA. Binding to IL-17RA at one side of the IL-17A molecule induces a conformational change in the second, symmetry-related receptor site of IL-17A. This change favors, and is sufficient to account for, the selection of a different receptor polypeptide to complete the cytokine-receptor complex. The structural results are supported by biophysical studies with IL-17A variants produced by site-directed mutagenesis. Cytokines of the interleukin-17 family promote the maintenance of both adaptive and innate immunity [1] , [2] , [3] , [4] , [5] , [6] , [7] , [8] , [9] , [10] , [11] . Dysregulation of their production may contribute to inflammatory and autoimmune diseases such as rheumatoid arthritis, psoriasis and asthma [1] , [2] , [12] , [13] , [14] . As such, they are attractive targets for therapeutic interventions [15] , [16] , [17] , [18] . The IL-17 cytokines are dimeric proteins: six homodimeric forms are designated IL-17A through IL-17F, and heterodimeric IL-17A/F is also known [19] , [20] . Five receptor polypeptides are named IL-17RA through IL-17RE. Convincing evidence shows that IL-17A, IL-17F and IL-17A/F require a heterodimeric receptor complex comprising IL-17RA and IL-17RC for signaling [19] , [20] , [21] , [22] , [23] , [24] , [25] . More generally, IL-17RA is shown to be a shared receptor for other IL-17 cytokines, with different receptor chains joining it in complex with the cytokines [2] , [3] , [8] , [22] , [23] , [26] , [27] , [28] , [29] , [30] . IL-17RA has high affinity for IL-17A, ~100-fold weaker affinity for IL-17F, and an intermediate affinity for the IL-17A/F heterodimer [19] , [20] , [21] , [22] . It has much weaker affinities for IL-17B, C, D and E [2] , [7] , [8] , [22] , [26] , [27] , [28] , [31] . In keeping with the general picture of how a cytokine is recognized by two different receptors (for example, IL-4 by IL-4Rα and γc) [32] , the interaction between an IL-17 and its primary receptor displays sufficiently high affinity to permit binding when the cytokine at physiological concentrations can diffuse freely relative to the membrane-bound receptor [2] , [3] , [8] , [22] , [23] , [26] , [27] , [28] , [29] , [30] , while a secondary receptor can be bound with more moderate affinity suited to an interaction that takes place in the two-dimensional space of the membrane [2] , [7] , [8] , [22] , [26] , [27] , [28] , [31] . The intermediate complex formed by an IL-17 and its primary receptor determines the exact binding surface presented to the secondary receptor. For IL-17 dimers, measured affinities indicate that this new binding surface must disfavor binding of the primary receptor, while creating features that favor binding of the secondary receptor. Overall, defining the structural features of intermediate and complete IL-17 complexes is a key to rationalizing the specificity inherent to the system as a whole [1] , [11] , [33] . Crystal structures are available for free IL-17F [21] , for IL-17A in complex with an antibody [34] , and for an IL-17F/IL-17RA complex [22] . In all these structures, the homodimeric cytokine displayed a cystine-knot fold with two intramolecular disulfides similar to that of nerve growth factor [35] . However, the important N-terminal region of IL-17A was disordered in the structure of the antibody complex [34] , and we demonstrate in this report that the mechanism by which the IL-17F/IL-17RA complex was suggested to disfavor binding of a second IL-17RA [22] is not supported by new structural data presented herein. In addition, as IL-17RC is the high affinity receptor for IL-17F [20] , [22] , [25] , the IL-17F/IL-17RA complex may not be the physiologically relevant intermediate complex of IL-17F. Nevertheless, the IL-17F/IL-17RA structure has given the first direct insight into the mode of binding, showing that the receptor binds the cytokine by engaging both its polypeptide subunits at their interface. More structures of IL-17 and detailed analysis have been needed, and we report herein two new structures that add greater detail to our understanding of how IL-17 and its receptors recognize each other. The first structure reported here is that of a free IL-17A homodimer in which the N terminus is more completely defined than in the previously solved antibody complex. The newly defined elements contribute to the structural integrity of the free homodimer. In the second structure, which is that of an IL-17A/IL-17RA intermediate complex, it becomes apparent that through an allosteric mechanism, conformational shifts in the same N-terminal elements strongly disfavor binding of a second molecule of IL-17RA. Similar allosteric effects appear to explain why IL-17F bound to one molecule of IL-17RA exhibits much weaker affinity for a second IL-17RA polypeptide. Supported by mutagenesis studies, our structures also provide a structural rationale for differences between the respective affinities of IL-17RA for different IL-17 cytokines. Generating suitable protein reagents for crystallizations Purification and crystallization of IL-17A (UniProtKB accession code Q16552) expressed in mammalian or insect cells can be complicated by heterogeneous post-translational protein modifications [7] , [19] , [20] , [21] , [34] , [36] . To avoid these problems, we expressed a recombinant IL-17A that lacked the first 10 N-terminal residues of the mature cytokine, and had two further mutations; these were N45D, to suppress N-glycosylation at the single canonical site, and C106S, to eliminate the free thiol group predicted to be exposed by elimination of its disulfide partner at C10. A construct encoding a precursor to this protein was expressed with good yield in mammalian cells, fully processed and secreted as the desired homodimeric product, and purified by standard methods. In surface plasmon resonance (SPR) measurements, its affinity ( K d =7 nM) for IL-17RA ECD was in the same range as that of recombinant wild-type IL-17A ( K d =1.3 nM). It crystallized readily. The amino-acid sequence of IL-17RA (UniProtKB accession code Q96F46) includes seven canonical sites for N-glycosylation. After it was found that a recombinant form of the protein expressed in insect cells was multiply glycosylated, two of the sites were mutated (N175D and N234D) and deglycosylation of IL-17RA at the remaining five sites was attempted using N-glycosidase F. LC-MS peptide mapping showed that N36 and N211 were successfully deglycosylated, but N18, N23 and N194 resisted complete deglycosylation. Mass spectrometry of N-glycopeptides in tryptic digests indicated that fucosylated oligomannose-3 glycans accounted for the great majority of sugar groups. Deglycosylated IL-17RA double mutant had essentially the same affinity for IL-17A as recombinant wild-type IL-17RA ( K d =1.9 nM versus 1.3 nM), and was free of aggregation. Using immobilized biotinylated IL-17A, only one binding event was observed in SPR between either the wild-type or mutant IL-17A and either wild-type or mutant IL-17RA, for concentrations of IL-17RA up to 150 nM. The IL-17A/IL-17RA complex sample used for crystallization ran in size-exclusion chromatography as a complex of IL-17A homodimer bound to a single IL-17RA molecule, even with total protein concentrations up to 9 mg ml −1 . Structure determination of IL-17A and its complex with IL-17RA Crystals of IL-17A diffract to 2.48 Å, and contain one IL-17A dimer in the asymmetric unit. 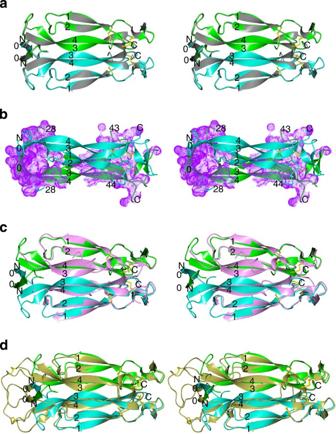Figure 1: Unbound IL-17A is highly symmetrical. (a) Wall-Eye stereo presentation of the overall structure of the unbound IL-17A dimer shown in ribbons (chain A, green; chain B, cyan), superimposed with its two-fold symmetry related dimer (gray). Least square superimposition was carried out using program LSQMAN45. The N- and C termini and the secondary structural elements are labeled. Disulfide bonds are shown as yellow sticks. The same coloring scheme is used throughout this report, unless otherwise noted. Molecular pictures are prepared using program PyMol46. (b) The distributions of inter-chain interactions (purple surface representing the dimerization interface) in the IL-17A dimer. For clarity, the IL-17A dimer is rotated 90 ° relative to A) to put chain B on top, and only the dimerization interface from chain A is shown. The gap in the 0–1 loop is also labeled. The dimerization interface was calculated using program PISA47. (c) Overlay of the unbound IL-17A with the antibody bound IL-17A (pink). (d) Overlay of the unbound IL-17F (gold) with IL-17A. The structure was determined by the molecular replacement method, and refined well without any Ramachandran outliers ( Table 1 ). Table 1 Data collection and refinement statistics. Full size table The IL-17A/IL-17RA complex crystals diffracted anisotropically to 2.9 Å along the c * axis and 3.3 Å in the perpendicular directions ( Table 1 ). The IL-17A/IL-17RA complex crystal structure was also determined by molecular replacement. The asymmetric unit of the complex crystal contains two copies of the IL-17A/IL-17RA 2:1 complex. In general, complex 1 (chains A, B and C) is more ordered than complex 2 (chains D, E and F). IL-17RA in complex 1 (chain C) can be modeled from residues 2–273 (numbering starts with the mature receptor), and residues 2–272 (chain F) are visible in the electron density in complex 2 ( Supplementary Fig. S1 illustrates electron density quality). All the predicted disulfide bonds in IL-17RA ECD can be built in both complexes. Electron densities for the remaining glycans were observed at N18, N23 and N194 of both IL-17RA molecules. In the following discussion, we concentrate mostly on complex 1 for structural analysis. Owing to poor electron densities in some areas, the final refined IL-17A/IL-17RA complex model has a few Ramachandran outliers ( Table 1 ). These outliers (residues 40 and 103–105 of IL-17A chains B and E) are located at the 0–1 and 3–4 loops of IL-17A (see below for structure descriptions). Unbound IL-17A homodimer is highly symmetric Two IL-17A monomers form a parallel dimer, and they are highly similar ( Fig. 1a ). The root mean square deviation (rmsd) from all Cα atom pairs in the dimer is 0.36 Å, and almost all side chains can be superimposed very well. Figure 1: Unbound IL-17A is highly symmetrical. ( a ) Wall-Eye stereo presentation of the overall structure of the unbound IL-17A dimer shown in ribbons (chain A, green; chain B, cyan), superimposed with its two-fold symmetry related dimer (gray). Least square superimposition was carried out using program LSQMAN [45] . The N- and C termini and the secondary structural elements are labeled. Disulfide bonds are shown as yellow sticks. The same coloring scheme is used throughout this report, unless otherwise noted. Molecular pictures are prepared using program PyMol [46] . ( b ) The distributions of inter-chain interactions (purple surface representing the dimerization interface) in the IL-17A dimer. For clarity, the IL-17A dimer is rotated 90 ° relative to A) to put chain B on top, and only the dimerization interface from chain A is shown. The gap in the 0–1 loop is also labeled. The dimerization interface was calculated using program PISA [47] . ( c ) Overlay of the unbound IL-17A with the antibody bound IL-17A (pink). ( d ) Overlay of the unbound IL-17F (gold) with IL-17A. Full size image Each IL-17A monomer contains a pair of anti-parallel β-sheets, one built from strands 1 and 2 and the second from strands 3 and 4 ( Fig. 1a ). The overall structure adopts a cystine-knot fold [35] . Consistent with the flexibility observed in the N terminus of antibody-bound IL-17A, each constituent monomer of the unbound IL-17A is disordered at the N terminus up to residue 18 and in the long connecting peptides 29–42. The two isolated peptides 19–28 form anti-parallel β-strands (strands 0); each runs parallel with strand 4 of the other monomer ( Fig. 1a ). Connections between strands 0 and the rest of the molecules are deduced from the IL-17A/IL-17RA complex structure discussed below, and are consistent with those of the unbound IL-17F structure. The C-terminal peptides 127–132 of IL-17A are disordered in both monomers. The N-terminal region of the unbound IL-17A dimer is less compact than its C-terminal region. Except for those involving strands 0, interchain interactions concentrate in its C-terminal region ( Fig. 1b ). The C-terminal region of the IL-17A is further rigidified by the presence of two intrachain disulfides in each subunit ( Fig. 1b ). The importance of strands 0 in the structural integrity of IL-17A dimer is supported by the failure of constructs lacking this sequence element to express properly in mammalian cells. Therefore, even though the N terminus of IL-17A is certainly more flexible than the C terminus, the interactions involving strands 0 appear to be essential contributors to maintaining a stable molecule. Comparison of the new structure for unbound IL-17A dimer with that of its antibody complex finds great similarity between the two (rmsd of 0.89 Å for 110 out of 147 pairs of Cα atoms). However, strands 0, parts of strands 3 and 4, and loop 3–4 are disordered in the antibody-bound IL-17A dimer ( Fig. 1c ). These peptides are well defined in the new structure, and they will be shown below to form the region that disfavors binding of a second IL-17RA molecule. Antibody-bound IL-17A was also very symmetric, with rmsd of 0.53 Å for all Cα atoms in the dimer. The structural match between the unbound IL-17A and IL-17F is better for the respective C-terminal regions than for the N termini (rmsd of 0.66 Å for 88 out of 166 pairs of Cα atoms in the dimer) ( Fig. 1d ). However, all β strands (0–4) are preserved between IL-17A and IL-17F. The unbound IL-17F dimer is also highly symmetric (rmsd of 0.43 Å from 110 out of 121 pairs of Cα atoms in each monomer), but two-fold symmetry breaks down at peptides 14–22 and 106–107, including the C17–C107 interchain disulfide, with deviations up to 3.5 Å. Overall structure of the IL-17A/IL-17RA complex As reported, the IL-17RA ECD contains two type III fibronectin domains, D1 and D2 [22] . The D1 domain of IL-17RA interacts with both chain A and chain B of IL-17A. IL-17RA D2 interacts mainly with IL-17A chain A ( Fig. 2a ). 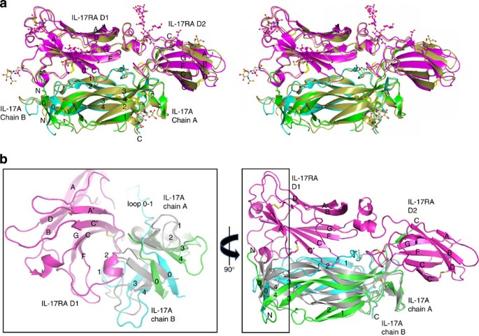Figure 2: Overall structure of the IL-17A/IL-17RA complex. (a) Wall-eye stereo presentation of the overall conformation that is conserved between IL-17A/IL-17RA (IL-17RA in magenta) and IL-17F/IL-17RA complex (both components gold). N-Glycosylation sites of the wild-type proteins are indicated by Asn side chains in ball-and-stick models, and by attached glycans when they were built in the models. Carbon atoms are colored according to their chains, and nitrogen and oxygen in blue and red, respectively. (b) IL-17RA binding induces large conformational changes in the IL-17A dimer. Right: the overview of the IL-17A/IL-17RA complex, with the unbound IL-17A dimer (gray) superimposed. Left: a zoomed-in view looking from strands 0. Figure 2: Overall structure of the IL-17A/IL-17RA complex. ( a ) Wall-eye stereo presentation of the overall conformation that is conserved between IL-17A/IL-17RA (IL-17RA in magenta) and IL-17F/IL-17RA complex (both components gold). N-Glycosylation sites of the wild-type proteins are indicated by Asn side chains in ball-and-stick models, and by attached glycans when they were built in the models. Carbon atoms are colored according to their chains, and nitrogen and oxygen in blue and red, respectively. ( b ) IL-17RA binding induces large conformational changes in the IL-17A dimer. Right: the overview of the IL-17A/IL-17RA complex, with the unbound IL-17A dimer (gray) superimposed. Left: a zoomed-in view looking from strands 0. Full size image The two IL-17A/IL-17RA complexes in the asymmetric unit have very similar overall structures, and all the Cα atom in the two complexes can be superimposed (rmsd value of 0.52 Å). They are also very similar to the IL-17F/IL17RA complex ( Fig. 2a ), with rmsd values of 1.1 Å and 0.89 Å when the maximum matching distances were set at 3.5 Å and 1.9 Å, respectively, in superimpositions (455 and 412 pairs of Cα atoms out of 469 in total, respectively). Based on these statistics, the maximum matching distance is set at 1.2 Å in all the following conformation analysis and modeling, to minimize inaccuracy in transformation matrix. The strands 0 and loops 0–1 and 3–4 in the cytokines, and loops A-B and D-F in IL-17RA domain D2 deviate significantly between the IL-17A/IL-17RA and IL-17F/IL-17RA complexes ( Fig. 2a ). Some of these differences are probably due to variations in crystal contacts. For example, the 3–4 loops of both cytokine chains in the IL-17A/IL-17RA complex are involved in crystal contacts, but this is not the case in the IL-17F/IL-17RA complex. The A–B and D–F loops of the IL-17RA D2 domain have different crystal contacts between IL-17A/IL-17RA and IL-17F/IL-17RA complexes. These deviating peptides do not locate at the binding interface ( Fig. 2a ). Other discrepancies are due to the sequence differences between IL-17A and IL-17F in strand 0 and loop 0–1. The IL-17RA/IL-17A complex structure was obtained using deglycosylated IL-17RA double mutant and truncated IL-17A. In contrast, the IL-17RA/IL-17F complex structure was obtained from fully glycosylated IL-17RA and full-length IL-17F with an intact interchain disulfide bond. Despite these differences, the two complexes share high overall similarity, supporting the view that the mutations and enzymatic deglycosylation do not disrupt IL-17RA interactions with IL-17A. Furthermore, no potential N-glycosylation site in any component of either the IL-17A/IL-17RA or IL-17F/IL-17RA complexes was located at a binding interface ( Fig. 2a ). The respective N termini of IL-17A and IL-17F are mostly disordered in both complexes. The interchain disulfide bond in IL-17F is disordered in its complex with IL-17RA. Binding to IL-17RA induces large conformational changes in the N-terminal region of the IL-17A dimer, but the C-terminal parts of both chains remain conformationally fixed. Because of these conformational changes, only 37 Cα atoms in chain A and 57 in chain B in the C-terminal half of the IL-17A dimer, superimpose well with the unbound IL-17A dimer (rmsd 0.58 Å). Relative to the unbound IL-17A, the entire N-terminal half of chain A bends away from IL-17RA ( Fig. 2b ). In chain B, strands 1–2 bend slightly toward IL-17RA, and the 1–2 and 3–4 loops move away from the A′–A and F–G loops of the D1 domain, respectively ( Fig. 2b ). In addition, both strands 0 move significantly, but maintain their interchain interactions ( Fig. 2b ). IL-17RA binding also displaces the loop 0–1 in chain B of IL-17A and makes it almost completely ordered; in contrast, this loop in chain A remains disordered ( Fig. 2b ). In the IL-17RA complex, the C-terminal peptide 127–131 of IL-17A chain A becomes ordered and forms a parallel β-sheet with strand G of the IL-17RA D2 domain. In IL-17A chain B, this peptide remains disordered ( Fig. 2a and b ). The N-terminal regions of IL-17F also undergo major conformational changes upon IL-17RA binding ( Supplementary Fig. S2 ). Because of these conformational changes, only 71 Cα atoms in chain A and 59 in chain B (out of 104 in each chain) superimpose well with the unbound IL-17F dimer (rmsd 0.59 Å). Conformational changes in the receptor-bound IL-17A allow it to avoid steric clashes with the A′–A, C–C′ and F–G loops of the IL-17RA D1 domain, while also forming several favorable interactions ( Fig. 2b ). Loops A′–A and F–G of IL-17RA may not be able to change conformation easily, being rigidified by numerous interactions within the IL-17RA molecule, including the C26–C95 disulfide ( Fig. 2a and b ). Specific interactions between IL-17A and IL-17RA As the global conformation of IL-17RA complex with IL-17A or IL-17F is conserved, side chain interactions are likely to account for differences in affinities of IL-17RA for different IL-17. Before the complex forms, symmetrical IL-17 homodimers have two equivalent potential IL-17RA binding sites. In contrast, the IL-17A/F heterodimer has two non-equivalent sites. IL-17RA binds IL-17A at one such site, interacting extensively with both monomers to bury a total of ~2220 Å 2 of surface area ( Fig. 3a ). 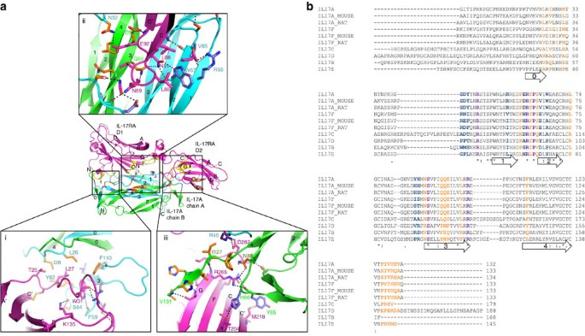Figure 3: Specific interactions of IL-17A with IL-17RA. (a) Overview mapping of the different regions of the complex interface onto the ribbon representations of IL-17A and IL-17RA, and their detailed views. Regions i, ii and iii are labeled in both the overview and the detailed views. In the overview, contacting residues in IL-17RA are colored yellow, and in IL-17A they are color coded according to sequence conservations: purple for residues conserved in all IL-17 members, orange for residues identical between IL-17A and IL-17F, and dark blue for residues unique to IL-17A. In the zoomed-in view panels, side chains and main chains engaged in interaction are shown in sticks and labeled. Carbon atoms of IL-17A side chains are colored according to their extent of sequence conservations. Hydrogen bonds are shown in dashes. (b) Sequence alignment of human, mouse and rat IL-17 highlighting interacting residues. Contacting residues in IL-17A/IL-17RA complex are color coded according to sequence conservations. Identical and conserved residues are also marked with ‘*’ and ‘:’ at the bottom of the sequences, respectively. Most IL-17RA interacting residues in IL-17A and IL-17F, respectively, are conserved across human, mouse and rat sequences. Strands 0–4 are indicated with empty arrows below their sequences. Figure 3: Specific interactions of IL-17A with IL-17RA. ( a ) Overview mapping of the different regions of the complex interface onto the ribbon representations of IL-17A and IL-17RA, and their detailed views. Regions i, ii and iii are labeled in both the overview and the detailed views. In the overview, contacting residues in IL-17RA are colored yellow, and in IL-17A they are color coded according to sequence conservations: purple for residues conserved in all IL-17 members, orange for residues identical between IL-17A and IL-17F, and dark blue for residues unique to IL-17A. In the zoomed-in view panels, side chains and main chains engaged in interaction are shown in sticks and labeled. Carbon atoms of IL-17A side chains are colored according to their extent of sequence conservations. Hydrogen bonds are shown in dashes. ( b ) Sequence alignment of human, mouse and rat IL-17 highlighting interacting residues. Contacting residues in IL-17A/IL-17RA complex are color coded according to sequence conservations. Identical and conserved residues are also marked with ‘*’ and ‘:’ at the bottom of the sequences, respectively. Most IL-17RA interacting residues in IL-17A and IL-17F, respectively, are conserved across human, mouse and rat sequences. Strands 0–4 are indicated with empty arrows below their sequences. Full size image Three IL-17RA-binding regions can be designated on the IL-17A homodimer: regions i and ii, formed by the N-terminal region and central β-strands of IL-17A, respectively, and each contacting the IL-17RA D1 domain; and region iii, where the C-terminal region of IL-17A contacts the IL-17RA D2 domain (see Fig. 3a for the overview of mapping of these regions and their detailed views. Also see Supplementary Fig. S3 for comparisons of these binding regions between IL-17A and IL-17F). To help in understanding the sequence specificity of IL-17A/IL-17RA interactions, the interacting residues are highlighted in a sequence alignment of IL-17 family members ( Fig. 3b ). At region i, the ends of strands 3 and 4, loop 1–2 and the beginning of loop 0–1 in chain B of IL-17A interact with loops A′–A and F–G of IL-17RA ( Fig. 3a ). Two major polar interactions, involving R101 of IL-17A and W31 of IL-17RA, are conserved in all IL-17 cytokines at this region ( Fig. 3a and b ). There is also an IL-17A- and IL-17F-specific water-mediated interaction at this region between S64 of IL-17A (S65 of IL-17F) and K135 of IL-17RA ( Fig. 3a ). An S65L mutant of IL-17F was recently identified in patients with impaired mucocutaneous IL-17 immunity against Candida albicans and Staphylococcus aureus [5] . Region ii, the major binding interface between IL-17A and IL-17RA, contains many specific hydrophilic interactions. Chain B of IL-17A contributes strands 1 and 2 and the C terminus of loop 0–1, and chain A contributes its strands 3 and 4. The C–C′ loop of the receptor D1 domain forms a majority of the interactions, with assistance from E127 on strand F ( Fig. 3a ). Among the residues at this region, D42, R55, V65 and W67 are unique to IL-17A, and N32, S40, Q94, E95 and L116 are identical between IL-17A and IL-17F ( Fig. 3b ). Region iii is mainly formed between the C-terminal region of IL-17A chain A and the D2 domain of IL-17RA ( Fig. 3a ). Among the residues that interact with IL-17RA, Y85 and H86 are unique to IL-17A at this site ( Fig. 3b ). The C-terminal peptide 127–131 in chain A of both IL-17A and IL-17F forms a parallel β-sheet with strand G of the receptor ( Fig. 3a and Supplementary Fig. S3 ). The sequence in peptide 127–131 is mostly conserved between IL-17A and IL-17F, but is divergent in other IL-17s. In summary, the higher affinity of IL-17RA for IL-17A compared with IL-17F is attributable to multiple interactions formed with the receptor that favor IL-17A over IL-17F. These are from cytokine chain B at region ii and chain A at region iii. When IL-17RA binds the IL-17A/F heterodimer at either of the two sites on the cytokine, it cannot have the favorable interactions that IL-17A homodimer achieves at both regions ii and iii, explaining the intermediate affinity with the heterodimer. Other interactions are common to IL-17A and IL-17F, but cannot be made by other IL-17 cytokines. Examples (using IL-17A numbering) are S64 at region i, E95 at region ii, and peptide 127–131 at region iii. The lack of these favorable interactions may weaken the affinities of IL-17B-E for IL-17RA. Mutagenesis studies of IL-17A The structural basis for the difference in affinity between IL-17A and IL-17F for IL-17RA was further probed by site-directed mutagenesis. IL-17A residues R55 and W67 at region ii and Y85 and H86 at region iii were each independently replaced by the corresponding residues in IL-17F, and the respective affinities for IL-17RA ECD of the four resulting IL-17A mutants (R55V, W67V, Y85I and H86S) were measured by SPR ( Fig. 4a ). Each mutation caused a 1.5–5.0-fold increase in K d relative to the recombinant wild-type cytokine ( Fig. 4b ). 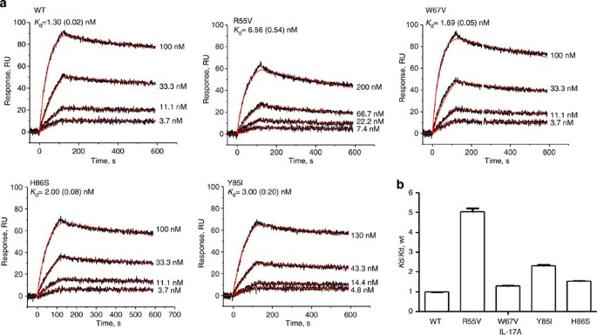Figure 4: Affinity of IL-17A for IL-17RA ECD measured by SPR. (a) Representative SPR sensorgrams (black lines) of the wild type, R55V, W67V, Y85I and H86S IL-17A binding to immobilized IL-17RA ECD in 10 mM HEPES, 150 mM NaCl, 0.005% p20, pH 7.4. Langmuir fits to the kinetic data are shown in red. Response (RU, resonance units) is plotted against time. Injected IL-17A concentrations are shown to right of the sensorgrams. (b) Fold difference in affinity caused by A/F residue substitutions. The affinity was based on average of six repeated kinetic experiments, with error bars representing one standard deviation. Figure 4: Affinity of IL-17A for IL-17RA ECD measured by SPR. ( a ) Representative SPR sensorgrams (black lines) of the wild type, R55V, W67V, Y85I and H86S IL-17A binding to immobilized IL-17RA ECD in 10 mM HEPES, 150 mM NaCl, 0.005% p20, pH 7.4. Langmuir fits to the kinetic data are shown in red. Response (RU, resonance units) is plotted against time. Injected IL-17A concentrations are shown to right of the sensorgrams. ( b ) Fold difference in affinity caused by A/F residue substitutions. The affinity was based on average of six repeated kinetic experiments, with error bars representing one standard deviation. Full size image Allosteric mechanism governing receptor complex composition In some ligand receptor complexes, binding of the first receptor presents a different high-affinity binding site for the second, identical receptor [37] . This does not happen in the case of IL-17A and IL-17F. The puzzle here is why a second IL-17RA cannot bind symmetrically to the IL-17A or IL-17F dimers, and achieve the same affinity as the first IL-17RA. Possible explanations include steric interference between two IL-17RA molecules in such a complex [22] , and/or conformational allosteric effects induced in the cytokine when it binds the first IL-17RA. To answer this question, we modeled the binding of a second IL-17RA molecule to the IL-17RA/IL-17A, using the two-fold rotational symmetry that relates two IL-17A monomers ( Fig. 5 ). We then checked which of the two mechanisms can account for the selection of IL-17A homodimer against the binding of a second IL-17RA. 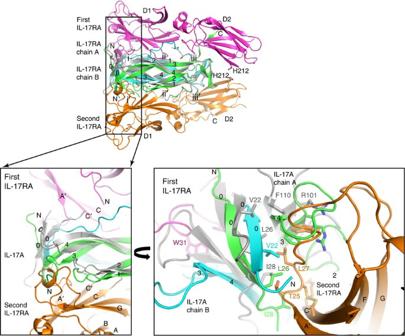Figure 5: IL-17A disfavors binding of a second IL-17RA through an allosteric mechanism. Top: a modeled IL-17RA/IL-17A/IL-17RA complex. The second IL-17RA (orange ribbons) is built from the first receptor through two-fold rotation relating the two IL-17A monomers. Superimposed with its two-fold rotation-related copy (gray), experimentally observed receptor bound IL-17A shows significant distortions of the two-fold symmetry at the N terminus, but remains symmetric at the C terminus. The binding regions on IL-17A for the first and the second IL-17RA are labeled i, ii, and iii, and i′, i′′ and i′′′ respectively. The only close contact between receptor 1 and 2 is at the side chains of H212 (stick model), at a distance of 4.2 Å. Bottom: zoomed-in views of the clashes between the second IL-17RA and IL-17A at region i′. Bottom right is a more detailed view with side chains of selected clashing residues shown in sticks. Side chains in gray indicate the optimal positions for interaction with the second IL-17RA. For simplicity, clashing residues involving loops 1–2 and 3–4 of IL-17A are not shown, because these loops might move freely. Figure 5: IL-17A disfavors binding of a second IL-17RA through an allosteric mechanism. Top: a modeled IL-17RA/IL-17A/IL-17RA complex. The second IL-17RA (orange ribbons) is built from the first receptor through two-fold rotation relating the two IL-17A monomers. Superimposed with its two-fold rotation-related copy (gray), experimentally observed receptor bound IL-17A shows significant distortions of the two-fold symmetry at the N terminus, but remains symmetric at the C terminus. The binding regions on IL-17A for the first and the second IL-17RA are labeled i, ii, and iii, and i′, i′′ and i′′′ respectively. The only close contact between receptor 1 and 2 is at the side chains of H212 (stick model), at a distance of 4.2 Å. Bottom: zoomed-in views of the clashes between the second IL-17RA and IL-17A at region i′. Bottom right is a more detailed view with side chains of selected clashing residues shown in sticks. Side chains in gray indicate the optimal positions for interaction with the second IL-17RA. For simplicity, clashing residues involving loops 1–2 and 3–4 of IL-17A are not shown, because these loops might move freely. Full size image Contrary to the earlier report [22] , we saw no steric clashes between two IL-17RA molecules ( Fig. 5 , top). The same modeling exercise showed that only the C-terminal half of the IL-17A dimer in IL-17RA complex obeys the native two-fold symmetry (rmsd 0.46 Å for 144 Cα pairs), and the N-terminal part of the IL-17A dimer deviates significantly ( Fig. 5 ). This structural asymmetry is caused by the large and different conformational changes required in each IL-17A polypeptide for binding to IL-17RA ( Fig. 2b ). Because of this structural asymmetry, region i′ (equivalent of region i for the second IL-17RA) on IL-17A is deformed and severe steric clashes would occur there if a second IL-17RA binds ( Fig. 5 , bottom). At region i′, the A′–A loop of a second IL-17RA D1 would clash with strands 3 and 4 of IL-17A chain A ( Fig. 5 , bottom left). Severe steric clashes are also observed at strands 0 for a second IL-17RA ( Fig. 5 , bottom right). When the first IL-17RA binds to IL-17A, these strands can move freely to avoid steric clashes ( Fig. 2b ). The same accommodation for a second IL-17RA is blocked by the first IL-17RA molecule already bound to IL-17A ( Fig. 5 , bottom). For residues that clash at region i′ ( Fig. 5 , bottom right), their symmetry-related mates form region i ( Fig. 3a ). None of these residues are near the glycosylation sites ( Fig. 2a ), and the mutations introduced in our samples should have minimal effects on the deformation of region i′. In the analysis above, only clashes involving residues in secondary structures of the IL-17A dimer are considered ( Fig. 5 ). These secondary structures (strands 0, 3 and 4) should be preserved ( Supplementary Fig. S4 ). Clashes involving loops 1–2 and 3–4 of IL-17A chain A at region i′ ( Fig. 5 ) might be avoidable if they could move freely. Region ii′ and iii′ do not seem to have any problem with the binding of a second IL-17RA. Consideration of the published IL-17F/IL-17RA complex structure indicates that the same allosteric mechanism also underpins the weak affinity of this complex for a second IL-17RA ( Supplementary Fig. S2 ). The C-terminal half of the IL-17F dimer (102 out of 171 pairs of Cα atoms) obeys the two-fold symmetry (rmsd 0.51 Å), and the N-terminal half deviates significantly. The single steric clash that appeared in the IL-17F/IL-17RA structure report (between two H212 side chains) [22] could be due to the inclusion of non-equivalent N-terminal residues in the IL-17F dimer in the determination of its two-fold symmetry. Nevertheless, it could be avoided easily by repositioning the exposed side chains. Analysis presented in this report addressed two aspects of the recognition of IL-17RA by IL-17 cytokines: the structural basis for the differences in affinity of IL-17RA for different cytokines and the molecular mechanism on which cytokine bound to one molecule of receptor has such sharply diminished affinity for a second receptor molecule of the same type. Thirteen residues are found to differ between IL-17A and IL-17F at their interfaces with IL-17RA ( Fig. 3b ), and they may account for ~100-fold higher affinity of IL-17A for the receptor than IL-17F. In structure-guided mutagenesis studies, four single-site mutations in IL-17A that replaced one residue with its IL-17F equivalent all reduced the affinity of IL-17A for IL-17RA. These four substitutions alone will account for ~22-fold difference in affinity between IL-17A and IL-17F for IL-17RA ( Fig. 4b and Supplementary Table S1 ). This analysis could have been further strengthened by mutagenesis experiments demonstrating potential increase in affinity when IL-17F residues are replaced with its IL-17A equivalents. The observations that IL-17RA adopts a conserved conformation in IL-17A and IL-17F complexes ( Fig. 2a ) and that some major IL-17RA interacting residues are identical among all IL-17 cytokines ( Fig. 3b ) support the view of IL-17RA as a shared receptor for other IL-17 cytokines [2] , [3] , [8] , [22] , [23] , [26] , [27] , [28] , [29] , [30] . IL-17RA may serve as a secondary receptor for IL-17B-F once these cytokines are captured by their primary receptors on the cell surface. Contrary to an earlier report [22] , an allosteric mechanism explains well why homodimeric IL-17A and IL-17F tend to disfavor binding of a second molecule of IL-17RA to their respective IL-17RA complexes. It remains less clear why IL-17A and IL-17F also select against two-fold binding of IL-17RC, but maintain reasonable propensities to co-bind IL-17RC and IL-17RA to form complete complexes [22] . The crystal structures of complexes with IL-17RC are needed. We can speculate that an IL-17RC complex, and more generally, other IL-17 receptor complexes, may use similar allosteric mechanisms to select IL-17RA over the same type of receptors. Protein constructs and expression For crystallization, a DNA construct of IL-17A double mutant (N45D/C106S) was made with the first 10 residues removed from the mature IL-17A, using standard PCR and QuikChangeII site-directed mutant genesis kit (Stratagen, CA, USA). This truncated, double mutant IL-17A construct was fused to a honeybee mellitin signal sequence and cloned into pCMV vector. IL-17A constructs with further truncations (20- and 34 N-terminal residues removed) were also made, but they did not express in HEK293 cells. For SPR studies, constructs of the full-length wild-type IL-17A and its R55V, W67V, Y85I and H86S single mutants were made with an N-terminal biotin acceptor peptide tag followed by a His 6 tag, using the native signal peptide for secretion. HEK293F cells were transfected with the DNA constructs using Freestyle Max Reagent (Invitrogen, NY, USA) according to the suggested protocols for expression. The ECD of IL-17RA used in this study, including the signal peptide, was cloned into a pFastBac vector with the carboxyl terminal fused to a thrombin cleavage site and a FLAG epitope. The DNA construct was transfected into Sf9 insect cells (Gibco) using Cellfectin II Reagent (Invitrogen) according to the suggested protocols for expression. To facilitate crystallization of the IL-17A/IL-17RA complex, a construct encoding N175D and N234D double mutant IL-17RA was expressed in similar fashion from insect cells. For SPR studies, the wild-type IL-17RA ECD was made. Protein purification The cultured cell media for the wild-type and IL-17A mutants were collected by centrifugation and the supernatant was filtered through a 0.22-μm filter. Ni-NTA Superflow resin was used for batch binding overnight. The resin was washed and then eluted with imidazole gradient in phosphate saline buffer (PBS, pH=7.4). Fractions containing IL-17A were pooled and further purified by size-exclusion chromatography on a Superdex75 column. Fractions containing properly dimeric IL-17A were pooled. For crystallization, the truncated IL-17A double mutant was concentrated to 10 mg ml −1 for crystallization using 10-kDa cutoff Vivaspin columns (GE LifeSciences, NJ, USA). The cultured cell medium for IL-17RA ECD was collected and filtered as above. Anti-FLAG antibody conjugate agarose (Sigma-Aldrich, MO, USA) resin was used for purification. Protein was eluted with 200 μg ml −1 FLAG peptide in PBS, dialyzed into PBS to remove FLAG peptide and then concentrated using Vivaspin columns. The concentrated IL-17RA protein was further treated with peptide N-glycosidase F (New England BioLabs, MA, USA) at 37 °C for 3 h. Deglycosylated IL-17RA was further purified on a size-exclusion Superdex 300 column equilibrated with PBS. The IL-17A/IL-17RA complex used for crystallization was generated by mixing enzymatic deglycosylated IL-17RA double mutant with slightly excess amount of truncated IL-17A. IL-17A/IL-17RA was separated from the unbound IL-17A on a Superdex 300 size-exclusion column equilibrated with PBS. Fractions containing the IL-17RA-IL-17A complex were concentrated to 9 mg ml −1 for crystallization trials. Crystallization and structure determination Both the unbound IL-17A and IL-17A/IL-17RA complex were crystallized using either sitting drop or hanging drop vapor diffusion methods. The crystallization of the unbound IL-17A was done at 22 °C. The crystallization drops were formed by mixing 1 μl of the truncated IL-17A at 10 mg ml −1 in PBS with 1 μl of well solution of 100 mM sodium citrate buffer, pH 5.0–6.0, 6–12% 2-propanol, and 10% w/v PEG10k. Crystals appeared in minutes and reached full sizes overnight. These unbound IL-17A crystals were soaked briefly in a cryo solution that consists of mother liquor plus 25% ethylene glycol before flashed cooled in liquid nitrogen. Crystallization of the IL-17A/IL-17RA complex was carried out at 22 or 4 °C. The complex at 9 mg ml −1 in PBS was mixed with a well solution of 0.1 M Tris HCl, pH 7.3–8, 20–25% Sokalan CP5 (Molecular Dimensions, Newmarket, UK). Crystals appeared overnight and grew to full size within a few days. Complex crystals were soaked briefly in a cryosolution consisting of the mother liquor plus 30% glycerol and flash cooled in liquid nitrogen. Data sets for both unbound IL-17A and IL-17A/IL-17RA complex crystals were collected at the APS IMCA 17-ID beamline (APS, Chicago, USA) and processed with program autoPROC [38] or HKL2000 [39] . Further data manipulations were carried out using the CCP4 program suite [40] . Structure determination was performed by molecular replacement with program PHASER [41] , using the IL-17A model in the antibody complex and IL-17F/IL-17RA as models for the unbound IL-17A and IL-17A/IL-17RA structures, respectively (PDB accession codes: 2VXS and 3JVF). Structure refinements were carried out with BUSTER with the TLS option [42] , [43] . During refinements, local structural similarity restraints were used, which greatly minimizes bias toward enforcing similarity in areas of real structural differences [43] . Manual model building was carried out with COOT [44] . Data collection and refinement statistics are listed in Table 1 . Surface plasmon resonance Surface plasmon resonance experiments were performed on a ProteOn XPR36 (BioRad, Hercules, CA). To enable the experiments with the WT and mutant IL-17A proteins, the receptor was first biotinylated by reaction with sulfo-NHS-LC-LC-biotin (Pierce) under stoichiometric conditions for 30 min at room temperature. Following the reaction, the sample was desalted to remove the excess biotin for capture. Receptor was then captured onto an NLC sensor chip to a level of ~200 RU. The running buffer for all SPR experiments was 10 mM HEPES, 150 mM NaCl, 0.005% p20. The WT and mutant IL-17A proteins used in these binding experiments were diluted in running buffer to the respective starting concentrations and serially diluted in three-fold increments. Proteins were loaded for 2 min over two receptor surfaces with dissociation times of 400 s. Because of the very slow off-rate for the proteins from the receptor, the surface was regenerated using a pulse of 3 M MgCl 2 after each injection. This regeneration step was shown to quantitatively remove IL-17A from the receptor. Proteins were run in triplicate over the two surfaces generating six individual sets of data for analysis. Data analysis was performed using the ProteOn analysis software. All data were fit to a simple 1:1 Langmuir binding model. Accession code: Coordinates and structure factors have been deposited into the Protein Data Bank under the accession codes 4HR9 (IL-17A) and 4HSA (IL-17A in complex with IL-17RA). How to cite this article: Liu Shenping et al. Crystal structures of interleukin 17A and its complex with IL-17 receptor A. Nat. Commun. 4:1888 doi: 10.1038/ncomms2880 (2013).